The condensin component NCAPG2 regulates microtubule–kinetochore attachment through recruitment of Polo-like kinase 1 to kinetochores The early event of microtubule–kinetochore attachment is a critical stage for precise chromosome segregation. Here we report that NCAPG2, which is a component of the condensin II complex, mediates chromosome segregation through microtubule–kinetochore attachment by recruiting PLK1 to prometaphase kinetochores. NCAPG2 colocalizes with PLK1 at prometaphase kinetochores and directly interacts with the polo-box domain (PBD) of PLK1 via its highly conserved C- terminal region. In both humans and Caenorhabditis elegans , when NCAPG2 is depleted, the attachment of the spindle to the kinetochore is loosened and misoriented. This is caused by the disruption of PLK1 localization to the kinetochore and by the decreased phosphorylation of its kinetochore substrate, BubR1. In addition, the crystal structure of the PBD of PLK1, in complex with the C -terminal region of NCAPG2, 1007 VLS-pT-L 1011 , exhibits structural conservation of PBD-phosphopeptides, suggesting that the regulation of NCAPG2 function is phosphorylation-dependent. These findings suggest that NCAPG2 plays an important role in regulating proper chromosome segregation through a functional interaction with PLK1 during mitosis. Chromosome condensation during mitosis is critical for proper bi-oriented chromosome separation [1] , [2] . The production of this mitosis-specific chromosome structure depends primarily on three multiprotein complexes: two condensin complexes and one cohesion complex [3] . Each condensin complex is composed of two ATPase subunit heterodimers (structural maintenance of chromosomes (SMC) 2 and 4) and three non-SMC regulatory subunits [2] , [3] . A unique set of three non-SMC regulatory components defines each condensin complex; NCAP-D2, NCAP-G and NCAP-H are parts of the condensin I complex, and NCAP-D3, NCAP-G2 and NCAP-H2 are components of the condensin II complex [2] , [3] , [4] . NCAPG and NCAPD2 in the condensin I complex and NCAPG2 and NCAPD3 in the condensin II complex are HEAT-repeat-containing regulatory subunits [5] . The condensin I complex, which has a conserved structure in both yeast and eukaryotes, is considered a canonical condensin complex functioning in eukaryotic chromosome condensation [2] . The condensin II complex regulates not only chromosome condensation but also a variety of cellular functions, including chromosome segregation, DNA repair, sister chromatid resolution, gene expression regulation and histone modulation [6] , [7] , [8] , [9] , [10] , [11] , [12] , [13] , [14] , [15] , [16] . Interestingly, homozygous mutants of all nematode condensin II complex components show nuclei with abnormal sizes or with an uneven distribution [11] . In human cells, depleting any condensin II complex component also results in defects in chromosome alignment or segregation [13] . The first step of chromosome segregation is microtubule attachment to the kinetochore on the chromosome [17] . The kinetochore is a protein complex assembly that corresponds to the centromere of the chromosome, where sister chromatids are linked [17] . Microtubule–kinetochore interactions require precise control to achieve the correct bi-orientation. The early event of microtubule attachment to the kinetochore before stabilizing the interactions is governed by Polo-like kinase 1 (PLK1) [17] , [18] , [19] , [20] , [21] . PLK1 localization changes based on the microtubule movements during mitosis, from the centrosome to the kinetochore and then to the midbody [18] , [20] , [22] . PLK1 localizes at the kinetochore until chromosome alignment is completed at the metaphase plate [18] . Until each kinetochore is properly occupied by a microtubule, PLK1 phosphorylates BubR1 and prevents the onset of anaphase [19] , [23] , [24] , [25] , [26] . Although some kinetochore proteins may be responsible for PLK1 localization at the kinetochore, further studies are required to identify the PLK1-regulating proteins that critically contribute to the role of PLK1 in microtubule-dependent chromosome alignment [17] . Interestingly, the condensin II complex localized at the kinetochore relative to the condensin I complex [13] , [27] , suggesting unique functional roles for these complexes during mitosis. However, the detailed mechanism of each condensin II complex component in chromosome segregation regulation remains unclear. In this study, we investigated the role of NCAPG2, which is a component of the condensin II complex, in chromosome segregation during mitosis using the nematode model Caenorhabditis elegans and a human cell line. Our results demonstrate that NCAPG2 contributes to chromosome segregation via microtubule–kinetochore attachment by mediating PLK1 localization at the kinetochore. This function of NCAPG2 is conserved in both nematodes and mammals and is essential for achieving chromosome integrity during cell division. NCAPG2 functions in the proper spindle attachment Although NCAPG2 has been less studied compared with NCAPD3, this subunit is predicted to play important roles similar to the other condensin subunits. To analyse the role of NCAPG2 in mitosis, we employed C. elegans , which is a simple metazoan that has a NCAPG2 homologue, capg-2 , and well-conserved condensin I and II complexes [11] . We depleted capg-2 expression using a bacteria-feeding RNA interference (RNAi) method. Consequently, chromosome segregation defects occurred in both germ cells and embryos ( Fig. 1a,b ), and these defects were similar to previously reported findings [11] . Proper chromosome segregation requires accurate orientation of the bipolar spindle attachment to the kinetochore, which is an early event [17] , [28] , [29] . Therefore, we examined CAPG-2 function when the microtubule–kinetochore dynamics were blocked by nocodazole, which interferes with microtubule polymerization. Nocodazole did not directly affect mitosis, and most embryos from the nocodazole-treated worms developed normally. However, combining the nocodazole treatment with capg-2 RNAi induced more severe defects during mitosis in early embryos than capg-2 RNAi alone ( Fig. 1b ). Moreover, the survival ratio of the progeny from adult worms after the sequential treatment of capg-2 RNAi feeding plus nocodazole was significantly reduced compared with the treatment with capg-2 RNAi feeding alone ( Fig. 1c ). This synergistic result suggests that CAPG-2 may function in the microtubule–kinetochore interaction during mitosis. Next, we observed the first cleavage process of embryos as a time course to determine the initial defect caused by CAPG-2 depletion during mitotic progression. Although chromosome condensation still occurred during mitosis, chromosome alignment at the metaphase plate was defective in CAPG-2-depleted embryos ( Fig. 1d ). Surprisingly, spindle attachment to the chromosome tended to be disoriented with capg-2 RNAi feeding ( Fig. 1e ). These results suggest that capg-2 is involved in the proper orientation of the spindle attachment to the chromosomes in C. elegans . 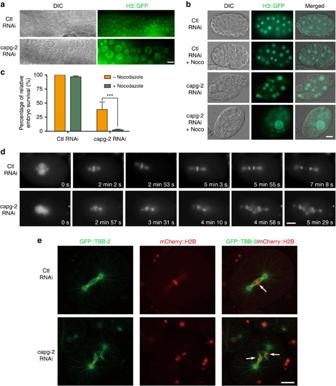Figure 1: Chromosomal segregation defects resulting from depletion of the condensin subunit CAPG-2 inC. elegans. (a) CAPG-2 depletion by RNAi resulted in abnormal germ cells. GFP-tagged H3 histone (HIS-72) showed large nuclei and extremely small nuclei in the gonads ofcapg-2RNAi-treated adult worms. Scale bar, 10 μm. (b) Combination ofcapg-2RNAi and nocodazole treatment showed severe abnormalities during embryonic cell division compared withcapg-2RNAi alone. Noco: nocodazole. Scale bar, 10 μm. (c) Quantitative analysis of embryonic survival after nocodazole treatment in either control or CAPG-2-depleted embryos. ***Pvalue fromt-test of nocodazole treatment compared with each control <0.001. Error bar, s.e.m.n=292, 245, 92 and 64, respectively, from the left. Three independent tests showed the same tendency. (d) Time-lapse images of chromosome segregation during mitosis with either control or CAPG-2 depletion. CAPG-2-depleted embryos had severe defects in chromosome alignment and segregation.C. elegansexpressing GFP::H2B (HIS-11) and GFP::TBB-2 depict the first cleavage at several time points in one-cell-stage embryos. Scale bar, 10 μm. (e) Chromosome alignments and uneven chromosome–microtubule attachment defects with CAPG-2 depletion inC. elegans. Abnormal chromosome alignment and segregation (red, H2B::mCherry (HIS-58); arrow) are shown at the first cleavage in an embryo aftercapg-2RNAi treatment. GFP::TBB-2 shows centrosomes and spindle fibres. Scale bar, 10 μm. Figure 1: Chromosomal segregation defects resulting from depletion of the condensin subunit CAPG-2 in C. elegans . ( a ) CAPG-2 depletion by RNAi resulted in abnormal germ cells. GFP-tagged H3 histone (HIS-72) showed large nuclei and extremely small nuclei in the gonads of capg-2 RNAi-treated adult worms. Scale bar, 10 μm. ( b ) Combination of capg-2 RNAi and nocodazole treatment showed severe abnormalities during embryonic cell division compared with capg-2 RNAi alone. Noco: nocodazole. Scale bar, 10 μm. ( c ) Quantitative analysis of embryonic survival after nocodazole treatment in either control or CAPG-2-depleted embryos. *** P value from t -test of nocodazole treatment compared with each control <0.001. Error bar, s.e.m. n =292, 245, 92 and 64, respectively, from the left. Three independent tests showed the same tendency. ( d ) Time-lapse images of chromosome segregation during mitosis with either control or CAPG-2 depletion. CAPG-2-depleted embryos had severe defects in chromosome alignment and segregation. C. elegans expressing GFP::H2B (HIS-11) and GFP::TBB-2 depict the first cleavage at several time points in one-cell-stage embryos. Scale bar, 10 μm. ( e ) Chromosome alignments and uneven chromosome–microtubule attachment defects with CAPG-2 depletion in C. elegans . Abnormal chromosome alignment and segregation (red, H2B::mCherry (HIS-58); arrow) are shown at the first cleavage in an embryo after capg-2 RNAi treatment. GFP::TBB-2 shows centrosomes and spindle fibres. Scale bar, 10 μm. Full size image To further examine the role of NCAPG2 in the microtubule–kinetochore interaction, we observed this interaction following treatment with monastrol, which is an Eg5 spindle motor protein inhibitor that effectively blocks the bipolarity of mitotic spindles in mammalian cells [30] . Similar to our previous observation in C. elegans , monastrol treatment resulted in deteriorated microtubule–chromosome interactions in NCAPG2-depleted MDA-MB-231 cells ( Fig. 2a ). These defective microtubule–kinetochore interactions resulted in complications during chromosome segregation. Centromere fluorescence in situ hybridization showed that NCAPG2-depleted cells treated with nocodazole possessed multiple centromeres compared with the control cells ( Fig. 2b,d ). For quantification, we counted the number of metaphase chromosomes in each cell. When NCAPG2 was depleted without nocodazole treatment, the population of cells containing more than 2 n (=46) chromosomes increased ( Fig. 2c ). Moreover, the number of cells containing 4 n (=92) or more chromosomes greatly increased in NCAPG2-depleted and nocodazole-treated cells ( Fig. 2e ). This aneuploidy resulting from NCAPG2 depletion is similar to the unusually large nuclei that formed in C. elegans when fed capg-2 RNAi. These findings suggest the involvement of NCAPG2 in the proper interaction between microtubules and kinetochores and, thus, critical roles for NCAPG2 during chromosome segregation in both nematode and mammalian cells. 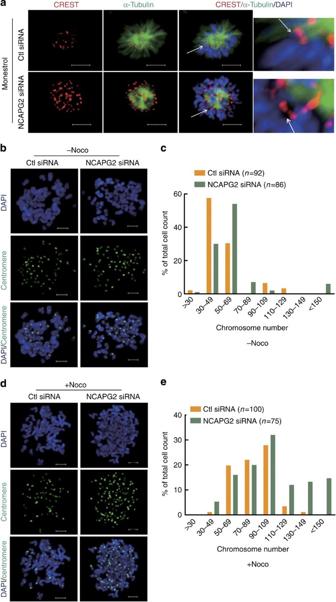Figure 2: NCAPG2 stabilizes microtubule–kinetochore interactions for proper chromosome segregation in human cells. (a) The integrity of microtubule attachments to chromosomes was visualized in monastrol-treated cells. Kinetochores and microtubule were visualized by staining with the anti-CREST antibody in either control or NCAPG2 siRNA-treated cells. Scale bar, 5 μm. Enlarged images of kinetochore–microtubule attachments were viewed in separate sections. (b) Images of centromere FISH signals and DAPI staining without nocodazole. (c) Distribution of the cell population according to the chromosome number per cell. Chromosome numbers were counted in vehicle-treated cells after metaphase spreading. Control siRNA-treated cells are presented as an orange bar and NCAPG2-depleted cells are presented as a green bar. (d) Images of centromere FISH signals and DAPI staining with nocodazole (50 ng ml−1). (e) Distribution of the cell population according to the chromosome number per cell. Chromosome numbers were counted in nocodazole (50 ng ml−1)-treated cells after metaphase spreading. Figure 2: NCAPG2 stabilizes microtubule–kinetochore interactions for proper chromosome segregation in human cells. ( a ) The integrity of microtubule attachments to chromosomes was visualized in monastrol-treated cells. Kinetochores and microtubule were visualized by staining with the anti-CREST antibody in either control or NCAPG2 siRNA-treated cells. Scale bar, 5 μm. Enlarged images of kinetochore–microtubule attachments were viewed in separate sections. ( b ) Images of centromere FISH signals and DAPI staining without nocodazole. ( c ) Distribution of the cell population according to the chromosome number per cell. Chromosome numbers were counted in vehicle-treated cells after metaphase spreading. Control siRNA-treated cells are presented as an orange bar and NCAPG2-depleted cells are presented as a green bar. ( d ) Images of centromere FISH signals and DAPI staining with nocodazole (50 ng ml −1 ). ( e ) Distribution of the cell population according to the chromosome number per cell. Chromosome numbers were counted in nocodazole (50 ng ml −1 )-treated cells after metaphase spreading. Full size image NCAPG2 functions in BubR1 kinetochore localization To examine the effect of NCAPG2 function on microtubule–chromosome interactions, we monitored the subcellular localization and phosphorylation of BubR1, which is one of the key kinetochore proteins mediating microtubule–kinetochore attachments [23] , [24] , [25] , [26] . From prometaphase to anaphase, BubR1 localizes at the kinetochore in a dumbbell-like manner [31] . Interestingly, the depletion of NCAPG2 clearly interferes with BubR1 localization at the kinetochore ( Fig. 3a ). We note that BubR1 phosphorylation by PLK1 at the kinetochore is important for facilitating proper interactions between chromosomes and microtubules [19] , [23] , [25] . Thus, we further examined the effect of NCAPG2 depletion on the functional interaction between BubR1 and PLK1 regarding kinetochore localization. Importantly, NCAPG2 depletion also disrupted PLK1 localization at the kinetochore ( Fig. 3b ). Furthermore, BubR1 phosphorylation at Ser676, which is a known substrate residue of PLK1, decreased in NCAPG2-depleted cells ( Fig. 3c ). These results indicate that NCAPG2 may be required for PLK1 recruitment to the kinetochore to allow the functional interaction with BubR1. 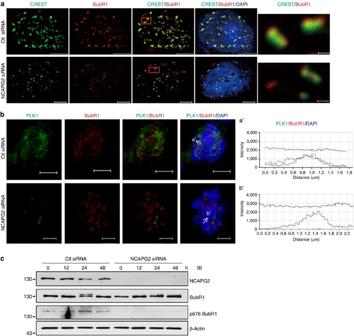Figure 3: NCAPG2 contributes to the PLK1–BubR1 interaction at kinetochores. (a) CREST and BubR1 were immunostained and visualized as pseudo-colour images obtained using a confocal microscope. Scale bar, 5 μm. Enlarged images in squares indicate BubR1 localization at the kinetochore end. Scale bar, 0.5 μm. (b) BubR1 and PLK1 were immunostained and visualized as pseudo-colour confocal microscope images of control or NCAPG2 siRNA-treated cells. The fluorescence intensity of each indicated spot was calculated from microscope images. Scale bar, 5 μm. (c) Immunoblotting of each indicated antibody was performed using either control GFP or NCAPG2 siRNA-treated cell lysates. Figure 3: NCAPG2 contributes to the PLK1–BubR1 interaction at kinetochores. ( a ) CREST and BubR1 were immunostained and visualized as pseudo-colour images obtained using a confocal microscope. Scale bar, 5 μm. Enlarged images in squares indicate BubR1 localization at the kinetochore end. Scale bar, 0.5 μm. ( b ) BubR1 and PLK1 were immunostained and visualized as pseudo-colour confocal microscope images of control or NCAPG2 siRNA-treated cells. The fluorescence intensity of each indicated spot was calculated from microscope images. Scale bar, 5 μm. ( c ) Immunoblotting of each indicated antibody was performed using either control GFP or NCAPG2 siRNA-treated cell lysates. Full size image NCAPG2 is required for PLK1 localization at the kinetochore Next, we examined whether the PLK1 recruitment to the kinetochore is directly regulated by NCAPG2. For this analysis, first, we examined the subcellular localization of NCAPG2 during mitosis. NCAPG2 was localized as nonspecific spreading in the nucleus during interphase ( Supplementary Fig. 1 ). In prometaphasic cells, NCAPG2 was spotted close to the kinetochore marker CREST ( Fig. 4a and Supplementary Fig. 1 ). The existence of NCAPG2 at the kinetochore exhibited similar spatial and temporal localization with PLK1 ( Fig. 4b and Supplementary Fig. 2 ). During metaphase, NCAPG2 disappeared from the kinetochore region of the aligned chromosomes but remained at the kinetochores of misaligned chromosomes ( Supplementary Fig. 1 ). During late-phase mitosis, NCAPG2 moved to the midzone and localized at the peripheral region of the midbody ( Supplementary Fig. 1 ). 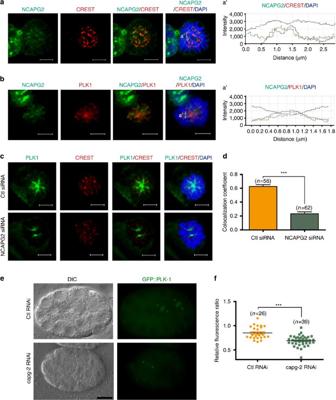Figure 4: NCAPG2 is required for PLK1 localization to kinetochores. (a) NCAPG2 and CREST images were detected from immunostaining, and their intensities were obtained from pseudo-colour confocal microscope images. Scale bar, 5 μm. (b) Immunostaining of NCAPG2 and PLK1 was detected using a microscope, and their intensities were calculated from the images. Scale bar, 5 μm. (c) Immunostaining of PLK1 and CREST was detected using a microscope, and their intensities were obtained from pseudo-colour images of either control or NCAPG2 siRNA-transfected cells. Scale bar, 5 μm. (d) Colocalization coefficients were calculated from the intensities of PLK1 and CREST images and represented as the mean±s.e. from the total sum of three independent experiments. ***Pvalue <0.001. (e) PLK1 localization was detected after control or CAPG-2 depletion using the transgenicC. elegansexpressing GFP::PLK-1 fusion protein. CAPG-2 depletion resulted in a decrease in GFP::PLK-1 at chromosomes, but not at centrosomes, inC. elegans. Scale bar, 10 μm. (f) Pseudo-colour images of GFP::PLK-1 fusion proteins were acquired. The intensities of GFP::PLK-1 at the kinetochore and centrosome were measured separately, and each ratio was calculated in each cell from either controls or CAPG-2-depleted cells usingC. elegansexpressing GFP::PLK-1. CAPG-2 depletion significantly reduced the level of GFP::PLK-1 at chromosomes. ***Pvalue <0.001. Figure 4: NCAPG2 is required for PLK1 localization to kinetochores. ( a ) NCAPG2 and CREST images were detected from immunostaining, and their intensities were obtained from pseudo-colour confocal microscope images. Scale bar, 5 μm. ( b ) Immunostaining of NCAPG2 and PLK1 was detected using a microscope, and their intensities were calculated from the images. Scale bar, 5 μm. ( c ) Immunostaining of PLK1 and CREST was detected using a microscope, and their intensities were obtained from pseudo-colour images of either control or NCAPG2 siRNA-transfected cells. Scale bar, 5 μm. ( d ) Colocalization coefficients were calculated from the intensities of PLK1 and CREST images and represented as the mean±s.e. from the total sum of three independent experiments. *** P value <0.001. ( e ) PLK1 localization was detected after control or CAPG-2 depletion using the transgenic C. elegans expressing GFP::PLK-1 fusion protein. CAPG-2 depletion resulted in a decrease in GFP::PLK-1 at chromosomes, but not at centrosomes, in C. elegans . Scale bar, 10 μm. ( f ) Pseudo-colour images of GFP::PLK-1 fusion proteins were acquired. The intensities of GFP::PLK-1 at the kinetochore and centrosome were measured separately, and each ratio was calculated in each cell from either controls or CAPG-2-depleted cells using C. elegans expressing GFP::PLK-1. CAPG-2 depletion significantly reduced the level of GFP::PLK-1 at chromosomes. *** P value <0.001. Full size image To examine whether NCAPG2 contributes to PLK1 recruitment to kinetochores, we measured the fluorescence intensity of PLK1 and CREST pseudocolour images. Anti-PLK1 and anti-CREST antibody immunostaining was performed and analysed in control and NCAPG2-depleted cells ( Fig. 4 ). When NCAPG2 expression was downregulated using small interfering RNA (siRNA), the correlation of the immunostaining intensity between PLK1 and CREST became lower than the control ( Fig. 4c,d ). Moreover, we confirmed the relationship between NGAPG2 expression and PLK1 localization using the in vivo C. elegans model ( Fig. 4e,f ). The PLK1 homologue in C. elegans , PLK-1 (fused with green-fluorescent protein (GFP)), was expressed simultaneously at holocentric chromosomes and centrosomes during metaphase [32] . However, in contrast with the centrosome, the GFP::PLK-1 signal was weakened at chromosomes in capg-2 -depleted embryos ( Fig. 4e,f ). We quantified the fluorescence intensity at chromosomes and centrosomes in metaphase cells containing either control or capg-2 RNAi. The relative fluorescence intensity ratio of GFP::PLK-1 in chromosomes compared with that in centrosomes was significantly reduced in capg-2 -depleted embryos ( Fig. 4f ). This result was consistent with the relative fluorescence ratio coefficient found in human cells ( Fig. 4d ), although the kinetochore structure of mammalian cells is quite different from that of C. elegans . However, PLK1 localization at the midzone and midbody during cytokinesis was not affected by NCAPG2 depletion ( Supplementary Fig. 3 ). These results suggest that NCAPG2 is a critical mediator of PLK1 localization at the kinetochore for the proper microtubule–kinetochore interactions. NCAPG2 interacts with PLK1 Because NCAPG2 plays a critical role in PLK1 recruitment at the kinetochore, we examined whether NCAPG2 interacts with PLK1. Immunoprecipitation assays performed using the glutathione S -transferase (GST)-tagged full-length PLK1 protein and the FLAG-tagged full-length NCAPG2 protein showed that these two proteins interact with each other ( Fig. 5a ). In addition, the incubation of FLAG-tagged NCAPG2 with the lysates of cells synchronized largely at prometaphase by nocodazole treatment showed that NCAPG2 forms a complex with endogenous PLK1 ( Fig. 5b ). To define the region of PLK1 that binds to NCAPG2, we designed various mutants of PLK1 ( Fig. 5c ). The immunoprecipitation assay showed that the polo-box domain (PBD) of PLK1 was responsible for the interaction with NCAPG2 ( Fig. 5d ). In addition, PBD domain mutants that included structural defects in the substrate-binding pocket (W414F, V415A, L427A; FAA) [33] did not bind to NCAPG2. 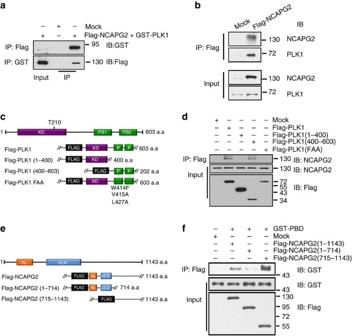Figure 5: PLK1 binding to NCAPG2 through the PBD. (a) Immunoprecipitation with FLAG or GST beads was performed in FLAG-NCAPG2- and GST-PLK1-transfected cells, and immunoblotting was conducted using reversed antibodies. (b) Detection of endogenous PLK1 binding to NCAPG2 was performed based on immunoprecipitation with FLAG beads in FLAG-NCAPG2-transfected cells. (c) Schematic of the PLK1 mutants for immunoprecipitation assay. KD: kinase domain, PB: polo-box domain. (d) Each PLK1 mutant was immunoprecipitated with FLAG beads, and NCAPG2 was detected with immunoblotting in each FLAG–PLK1 mutant-transfected cell. Each FLAG–PLK1 mutant-transfected cell was subjected to immunoprecipitation using FLAG beads, and NCAPG2 was detected by immunoblotting. (e) Schematic of the NCAPG2 deletion mutants forin vitroimmunoprecipitation assay. Rb: Rb binding motif, HEAT: HEAT repeat. (f) Purified GST-PBD was mixed with purified Flag-NCAPG2 fragments and pulled down. Bound GST–PBD was detected by immunoblotting. Figure 5: PLK1 binding to NCAPG2 through the PBD. ( a ) Immunoprecipitation with FLAG or GST beads was performed in FLAG-NCAPG2- and GST-PLK1-transfected cells, and immunoblotting was conducted using reversed antibodies. ( b ) Detection of endogenous PLK1 binding to NCAPG2 was performed based on immunoprecipitation with FLAG beads in FLAG-NCAPG2-transfected cells. ( c ) Schematic of the PLK1 mutants for immunoprecipitation assay. KD: kinase domain, PB: polo-box domain. ( d ) Each PLK1 mutant was immunoprecipitated with FLAG beads, and NCAPG2 was detected with immunoblotting in each FLAG–PLK1 mutant-transfected cell. Each FLAG–PLK1 mutant-transfected cell was subjected to immunoprecipitation using FLAG beads, and NCAPG2 was detected by immunoblotting. ( e ) Schematic of the NCAPG2 deletion mutants for in vitro immunoprecipitation assay. Rb: Rb binding motif, HEAT: HEAT repeat. ( f ) Purified GST-PBD was mixed with purified Flag-NCAPG2 fragments and pulled down. Bound GST–PBD was detected by immunoblotting. Full size image Next, we attempted to identify the region of NCAPG2 that binds to PLK1. An in vitro immunoprecipitation experiment using purified GST-PBD (371–594; bacterial expressed) and purified Flag-NCAPG2 (full length, N -terminal (1–714) or C -terminal NCAPG2 (715–1143); mammalian cell expressed) showed that the C -terminal region of NCAPG2 strongly binds to GST-PBD ( Fig. 5e,f ). These results suggest that the PBD of PLK1 interacts with the C -terminal region of NCAPG2. Given that the PBD of PLK1 preferentially binds to a strictly conserved serine residue followed by a phosphorylated serine or threonine residue (S-pS/T motif) for its proper targeting during mitosis [34] , we examined whether an S-pS/T motif exists in the C- terminal region of NCAPG2. Thr1010 and the surrounding residues of NCAPG2 are highly conserved from nematodes to mammals ( Fig. 6a ). We also confirmed the phosphorylation of this residue ( Supplementary Fig. 4 ). When Thr1010 was replaced with alanine, the PLK1 interaction significantly decreased ( Fig. 6a,b ). The phosphorylated peptide ( 1006 GVLS-pT-LI 1012 ) interacts strongly with the PBD of PLK1, with a K d value of 69.91±15.95 nM, which was obtained from a fluorescence polarization in vitro binding assay using synthetic peptides ( Fig. 6b ). We also determined the crystal structure of the PBD of PLK1 in complex with the 5-mer phosphopeptide 1007 VLS-pT-L 1011 at a resolution of 1.7 Å ( Fig. 6c , Table 1 and Supplementary Fig. 5 ). The PBD structure shows the typical architecture that has been previously reported [35] , [36] , [37] , [38] . Several antiparallel β-sheets from the two PBDs generate a shallow cavity that allows substrate binding. In adiition, the overall conformation of substrate peptides was conserved ( Fig. 6d ). The phosphothreonine residue (pT1010) forms hydrogen bonds with His538 and with Lys540, similar to other PBD-phosphopeptide structures ( Fig. 6d,e ) [35] , [36] , [38] . The binding mode of the peptide to the PBD of PLK1 is highly similar to that of other PBD–phosphopeptide complexes ( Fig. 6e ). 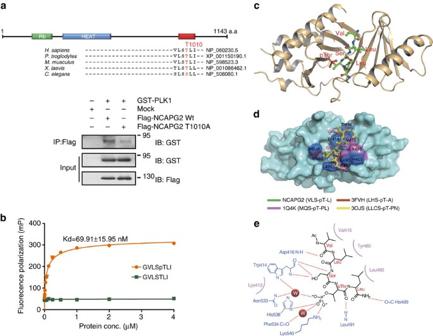Figure 6: Thr1010 of NCAPG2 is a critical binding motif for the PBD. (a) Scheme illustrating the possible binding motif for the PBD in the C-terminus of NCAPG2. Immunoprecipitation of FLAG-tagged wild-type or T1010A NCAPG2 mutants using GST-tagged PLK1 is also shown. (b) Results of fluorescence polarization for monitoring the binding of fluorescein isothiocyanate‐labelled peptides to the PBD of PLK1. The 1010pT peptide is shown in orange, and the non-phosphorylated 1010 peptide is shown in green. The data are presented as the mean±s.d. of triplicates of three independent experiments. (c) Crystal structure of the PBD in complex with the 1010pT peptide. The 1010pT peptide binds to the shallow cavity formed by the interface of the two PBs. (d) The superimposed view of PBD–phosphopeptide complexes. The PBD-1010pT peptide (PDB entry: 4O9W) is labelled in red and drawn in green, the PBD-PBIP peptide (PDB entry: 3FVH) is drawn in orange, the PBD-synthetic optimal peptide (PDB entry: 1Q4K) is drawn in pink and the PBD-Cdc25C peptide (PDB entry: 3OJS) is drawn in yellow. The residues of PBD that interact with the 1010pT peptide through hydrogen bonds or through hydrophobic contacts are labelled in black and represented in blue or in pink, respectively. (e) Schematic diagram of the 1010pT peptide-binding mode. ‘W’ represents a water molecule. Figure 6: Thr1010 of NCAPG2 is a critical binding motif for the PBD. ( a ) Scheme illustrating the possible binding motif for the PBD in the C-terminus of NCAPG2. Immunoprecipitation of FLAG-tagged wild-type or T1010A NCAPG2 mutants using GST-tagged PLK1 is also shown. ( b ) Results of fluorescence polarization for monitoring the binding of fluorescein isothiocyanate‐labelled peptides to the PBD of PLK1. The 1010pT peptide is shown in orange, and the non-phosphorylated 1010 peptide is shown in green. The data are presented as the mean±s.d. of triplicates of three independent experiments. ( c ) Crystal structure of the PBD in complex with the 1010pT peptide. The 1010pT peptide binds to the shallow cavity formed by the interface of the two PBs. ( d ) The superimposed view of PBD–phosphopeptide complexes. The PBD-1010pT peptide (PDB entry: 4O9W) is labelled in red and drawn in green, the PBD-PBIP peptide (PDB entry: 3FVH) is drawn in orange, the PBD-synthetic optimal peptide (PDB entry: 1Q4K) is drawn in pink and the PBD-Cdc25C peptide (PDB entry: 3OJS) is drawn in yellow. The residues of PBD that interact with the 1010pT peptide through hydrogen bonds or through hydrophobic contacts are labelled in black and represented in blue or in pink, respectively. ( e ) Schematic diagram of the 1010pT peptide-binding mode. ‘W’ represents a water molecule. Full size image Table 1 Data collection and refinement statistics. Full size table Trp414, which plays important roles in centrosome localization and in substrate binding without affecting kinase activity [22] , forms multiple hydrogen bonds with the serine residue of the substrate peptide in a direct or water-mediated manner. Moreover, many water molecules found near the phosphothreonine residue form a hydrogen bond network and strengthen the binding affinity, similar to PBD-Cdc25C-primed peptide structures [38] . A water molecule-mediated hydrogen bond network was formed by Trp414, Asn533 and the oxygen atom of phosphate. In addition, another water molecule forms a hydrogen bond with the carbonyl oxygen of Phe534 and with the oxygen atom of the phosphate in the substrate peptide. In addition, Asp416, His489 and Leu491 also participate in forming hydrogen bonds, and Lys413, Val415, Tyr485 and Leu490 form hydrophobic contacts with the 1010pT peptide. Interestingly, the CL loop, which connects the two PBs (residue 493–507) [38] and which is usually activated upon phosphopeptide binding, was partially disordered in our structure. As the Thr1010 position in NCAPG2 was critical for PLK1 binding, we performed reconstitution experiments after NCAPG2 siRNA transfection. For these experiments, we constructed siRNA resistant-based lentiviral vectors, wild-type or T1010A mutants of NCAPG2 (NCAPG2 R-Wt or NCAPG2 R-T1010A ). When NCAPG2 was depleted, PLK1 localization to the kinetochore disappeared. In contrast to wild-type NCAPG2, which rescued PLK1 localization to the kinetochore, the T1010A mutant was not able to recover PLK1 localization to the kinetochore ( Fig. 7a ). The relative fluorescence intensities of the PLK1 signal compared with the CREST signal were measured in the kinetochore after reconstitution. Compared with wild type, NCAPG2 R-T1010A failed to properly recruit PLK1 to the kinetochore ( Fig. 7b ). In addition, phosphorylated BubR1, which is shown as a band-shift, became diminished after nocodazole treatment in the T1010A mutant NCAPG2 was reconstituted ( Fig. 7c ). These results suggest that the NCAPG2 Thr1010 residue and its surrounding region in NCAPG2 are critical for PLK1 localization and function at the kinetochore. 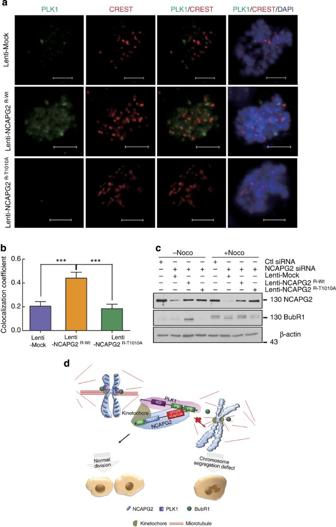Figure 7: NCAPG2 Thr1010 is required for PLK1 recruitment to kinetochores. (a) Lentivirus expressing the siRNA-resistant mock, wild-type or T1010A mutant NCAPG2Rinfected in NCAPG2 siRNA-transfected cells. PLK1 and CREST stained in wild-type or T1010A NCAPG2Rmutated lentiviral reconstituted cells. Scale bar, 5 μm. (b) Colocalization coefficients were calculated from the intensities of PLK1 and CREST staining in mock, wild-type or T1010A NCAPG2Rlentiviral reconstituted cells and represented as the mean±s.e. of the total sum of three independent experiments. (c) Immunoblotting performed after the reconstitution experiment using lentiviral wild-type or T1010A NCAPG2Rmutant expression with the indicated antibodies. (d) Model of NCAPG2 and PLK1 binding at kinetochores for proper microtubule–kinetochore assembly. In the presence of NCAPG2, PLK1 is recruited to the kinetochore and it phosphorylates BubR1, the PLK1 substrate at the kinetochore, which is required for precise chromosome segregation. Surveillance of proper microtubule–kinetochore assembly is activated, and microtubule–kinetochore attachments are fully satisfied before segregation. However, without NCAPG2, PLK1 localization and BubR1 phosphorylation are disrupted at the kinetochore. Therefore, NCAPG2 is necessary for proper PLK1 recruitment to the kinetochore and for precise chromosome segregation. Figure 7: NCAPG2 Thr1010 is required for PLK1 recruitment to kinetochores. ( a ) Lentivirus expressing the siRNA-resistant mock, wild-type or T1010A mutant NCAPG2 R infected in NCAPG2 siRNA-transfected cells. PLK1 and CREST stained in wild-type or T1010A NCAPG2 R mutated lentiviral reconstituted cells. Scale bar, 5 μm. ( b ) Colocalization coefficients were calculated from the intensities of PLK1 and CREST staining in mock, wild-type or T1010A NCAPG2 R lentiviral reconstituted cells and represented as the mean±s.e. of the total sum of three independent experiments. ( c ) Immunoblotting performed after the reconstitution experiment using lentiviral wild-type or T1010A NCAPG2 R mutant expression with the indicated antibodies. ( d ) Model of NCAPG2 and PLK1 binding at kinetochores for proper microtubule–kinetochore assembly. In the presence of NCAPG2, PLK1 is recruited to the kinetochore and it phosphorylates BubR1, the PLK1 substrate at the kinetochore, which is required for precise chromosome segregation. Surveillance of proper microtubule–kinetochore assembly is activated, and microtubule–kinetochore attachments are fully satisfied before segregation. However, without NCAPG2, PLK1 localization and BubR1 phosphorylation are disrupted at the kinetochore. Therefore, NCAPG2 is necessary for proper PLK1 recruitment to the kinetochore and for precise chromosome segregation. Full size image Condensin complexes have pivotal functions during mitotic chromosome condensation [2] . Although the role of the condensin complexes in chromosome segregation is highly conserved from nematodes to mammals [11] , [12] , [13] , [14] , little is known concerning the specific components of the condensin I or II complex that drive chromosome segregation and how these components function in the diverse steps of chromosome segregation. PLK1 localization at the kinetochore is essential for microtubule–kinetochore attachments and for reliable chromosome segregation [39] , [40] , [41] , [42] . In this study, we have shown that NCAPG2, which is one of the components of the non-SMC condensin II complex, may contribute to chromosome segregation by recruiting PLK1 to the kinetochore during prometaphase. To investigate the role of NCAPG2 in chromosome segregation, we used C. elegans and human cells as model systems ( Figs 1 and 2 ). When CAPG-2 was depleted in C. elegans , chromosome condensation occurred normally during early mitosis; however, chromosome alignment at the metaphase plate was delayed, and the chromosome was replicated again without cytokinesis ( Fig. 1d ). Interestingly, abnormal chromosome alignment by treatment with capg-2 -feeding RNAi was caused by a dispersed orientation of the microtubule attachment ( Fig. 1e ). CAPG-2 depletion caused defects in the proper interaction between microtubules and the kinetochore during early mitosis, resulting in chromosome missegregation. However, these types of defects resulting from CAPG-2 depletion did not occur when other condensin components were depleted in C. elegans [14] , [43] . Depletion of the condesin I complex component CAPG-1 occurs in the C. elegans chromosome segregation defect caused by Aurora B AIR2 -dependent chromosome obstruction [43] . CAPG-1 depletion results in cytokinesis failure, which is characterized by anaphase bridge formation [43] . Moreover, a temperature-sensitive mutant of another component of the condensin II complex, HCP-6 (NCAPD3 homologue in C. elegans ), also shows chromosome segregation defects. However, this non-functional hcp-6 mutant shows merotelic kinetochore–microtubule interactions caused by a failure to maintain chromosome rigidity [14] . The kinetochore–microtubule interaction defects observed in C. elegans are also observed in human cells ( Figs 1 and 2 ). Consistent with previous observations, siRNA-mediated depletion of condensin II components in HeLa cells causes defects in chromosome segregation [13] . NCAPD3 also plays a role in PLK1 localization to the chromosomal axes [44] . These results suggest that two individual condensin II components independently recruit PLK1 to different chromosome regions. These NCAPD3 affects on PLK1 during mitosis could explain our observation that the NCAPG2 T1010A mutant still had weak binding to PLK1, although the NCAPG2–PBD interaction was completely abolished when NCAPG2 was unphosphorylated at Thr1010, suggesting indirect binding through the condensin II complex ( Fig. 6a,b ). Condensin II complex localization at the centromere and at the chromosome arm is important for chromosome function during mitosis [13] . Mitotic chromosome condensation, which is governed by condensin complex proteins, is necessary for the proper centromere structure for kinetochore complex assembly [9] . We found in this study that NCAPG2 also has an additional role in proper microtubule attachment to the kinetochore via PLK1 for proper chromosome segregation [42] , [45] . Other proteins may be involved in PLK1 localization and delocalization to the kinetochore; PBIP1, BUB1, NUDC, INCENP and CUL3–KLHL22 may contribute cooperatively with or independent of NCAPG2 (refs 40 , 41 , 42 , 46 , 47 ). However, considering the depletion phenotypes, NCAPG2 plays the most critical role in the kinetochore–microtubule interaction governed by PLK1 during prometaphase to metaphase [40] , [41] , [46] , [47] , [48] . Taken together, NCAPG2 contributes to PLK1 kinetochore localization for the kinetochore–microtubule interaction, and CUL3–KLHL22 delocalizes PLK1 from the kinetochore after BubR1 phosphorylation [47] . These results suggest that PLK1 localization to the kinetochore is governed by different proteins and depends on the timeline of mitosis progression [40] , [47] . NCAPG2-regulated PLK1 localization occurs during the initial stage of the microtubule–kinetochore interaction because the NCAPG2 and PLK1 interactions primarily occur during prometaphase, before chromosome alignment is completed. In addition, our results showed that NCAPG2 is critical for PLK1 kinetochore localization in both human and nematode cells ( Fig. 3b and 4c–f ), suggesting functional conservation of NCAPG2 in nematodes and vertebrates. Therefore, we hypothesised that the PBD-binding site may be conserved across species and found a conserved PBD-recognition region at the C-terminus of NCAPG2 ( Fig. 6a ). In human NCAPG2, the PBD-recognition region was 1007 VLSpTLI 1012 , and C. elegans contained a similar sequence, 995 SLSpSLL 1000 . The peptide in C. elegans is relatively conserved within −2 to +2 amino-acid position with the human peptide; however, the threonine is replaced with serine. This region is highly conserved in other species, including Pan troglodytes and Xenopus laevis , indicating that the role of NCAPG2 in PLK1 localization to the kinetochore may be conserved ( Fig. 6a ). Our immunoprecipitation and in vitro binding assay data indicated that NCAPG2 and PLK1 directly interact with each other in a phosphorylation-dependent manner at Thr1010 ( Fig. 6a,b ). We confirmed that Thr1010 could be phosphorylated during mitosis by using a phosphospecific antibody ( Supplementary Fig. 4 ). In this study, we also determined the crystal structure of PLK1–PBD in complex with NCAPG2 phosphopeptides. This structure provides a detailed view of the interactions between PLK1 and NCAPG2. In addition, our structure provides another opportunity for developing PLK1 inhibitors that target the PBD. Many extensive studies have been established to develop PLK1 inhibitors that target the PBD [49] , [50] , [51] . These studies were initiated from structural investigations of the PBD and PBIP peptide structures [37] . As the peptide sequence from NCAPG2 is quite different from PBIP peptides, except for the characteristic S-pT residues, our structure will lay the groundwork for further developing PLK1 inhibitors. In summary, we found that NCAPG2 is a new critical player in PLK1 kinetochore localization. NCAPG2 interacts with PLK1 during the prometaphase–metaphase transition in unstable microtubule–kinetochore interactions. We suggest a model of NCAPG2 and PLK1 binding at the kinetochore for proper microtubule–kinetochore assembly ( Fig. 7d ). NCAPG2 localization and PLK1 recruitment to the kinetochores of misaligned chromosomes are critical for the completion of proper chromosome alignment at the metaphase plate. Our study suggests that the conserved function of NCAPG2 is essential for PLK1 localization to kinetochores and for proper chromosome segregation. C. elegans strains and RNA interference C. elegans were cultivated on NGM plates at 20 °C as a standard culture method [52] . The capg-2 RNAi clone was obtained from Dr J. Ahringer’s bacteria-feeding RNAi library, which was a kind gift from Dr J. Lee (Seoul National University). The wild-type N2 strain was used for measuring embryo lethality when capg-2 RNAi was treated with nocodazole. RW10006 (HIS-72::GFP), XA3501 (GFP::HIS-11 and GFP::TBB-2), JG479 (NPP-1::GFP, mCherry::HIS-58 and GFP::TBB-2) and SA127(GFP::PLK-1) were used to determine the effects of capg-2 knockdown on mitosis. JG479 was generated by crossing XA3501 and OCF3 (NPP-1::GFP and mCherry::HIS-58). HIS-72 is histone 3, and TBB-2 is β-tubulin. Both HIS-11 and HIS-58 are histone 2B proteins ( www.wormbase.org ). Most strains were provided by the CGC, which is funded by the NIH Office of Research Infrastructure Programs (P40 OD010440). For capg-2 RNA interference, L4 worms were transferred to the RNAi plate, and the F1 embryos were observed. The HT115 Escherichia coli strain, which contains the empty RNAi vector (L4440), was used as the control. To compare the survival ratios of embryos when capg-2 RNAi was treated with or without nocodazole, L4 worms were grown in liquid with or without nocodazole for 12 h after feeding on the capg-2 RNAi or control plates for 12 h. Next, the worms were recovered on NGM plates, and three adult worms were transferred to NGM plates. The worms were removed after laying eggs for 12 h, and the dead embryos were counted the next day. We examined three plates for each case, and all repeated tests showed the same tendency three times. The liquid culture used in the 96-well plates contained E. coli (OP50) and cholesterol, and the culture volumes were 100 μl each of nocodazole (20 μg ml −1 ) and 1% DMSO (control). All images of C. elegans embryos were observed and captured using an Imager A2 compound microscope (Carl Zeiss) or an LSM700 confocal microscope (Carl Zeiss). Experimental conditions MDA-MB-231 and HEK293 cells, which were purchased from the American Type Culture Collection, were grown in Dulbecco’s modified Eagle’s media (Invitrogen) supplemented with 10% fetal bovine serum (Invitrogen) and 1% penicillin–streptomycin (P/S) in a 5% CO 2 atmosphere at 37 °C. siRNAs for NCAPG2 were synthesised using 5′-GCUUCAUAGGGUCAUUUAUTT-3′ and 5′-GAAGAAUGAUGCUGAAACATT-3′ sequences (ST Pharm. Co. LTD). Expression vectors or siRNAs were transferred into the cells using the Amaxa Nucleofector system (Amaxa Biosystems) according to the manufacturer’s instructions. For synchronizing cells into a specific phase, 50 ng ml −1 nocodazole (Sigma-Aldrich) or 100 μM monastrol (Sigma-Aldrich) was used. Immunofluorescence imaging Cell were grown on coverslips, rinsed twice with PHEM buffer (60 mM PIPES, 25 mM HEPES, 10 mM EGTA and 2 mM MgCl 2 , pH 6.9 with KOH), permeabilized with 0.5% Triton X-100 in PHEM buffer at 4 °C for 1 min and fixed with 4% paraformaldehyde in PHEM buffer. The fixed cells were incubated at 4 °C for 1 h with each primary antibody, followed by incubation with a secondary antibody plus 100 ng ml −1 4',6-diamidino-2-phenylindole (DAPI) for 3 h. The acquired images were analysed using a confocal microscope (Zeiss 510 Meta, Carl Zeiss). Counting the chromosome number Cells were harvested after 4 h colcemid (0.1 μg ml −1 ) treatment with or without nocodazole (50 ng ml −1 ) pretreatment. The harvested cells were incubated with a hypertonic solution (0.075 M KCl) and with freshly prepared fixative (methanol/acetic acid, 3:1). The swollen cells were spread on a glass slide. The slides were dried at room temperature, stained with DAPI (100 ng ml −1 ) and visualized under a confocal microscope. Vector construction and site-directed mutagenesis The NCAPG2 expression vectors were constructed using pcDNA3.1 , pCMV-3FLAG-1 and pLL3.7 vectors with KpnI/XhoI, EcoRV/XhoI and SmaI/XhoI restriction enzyme sites, respectively. To produce siRNA-resistant NCAPG2 mutants (Lenti-NCAPG2 R ), the mutants (forward primer: 5′-GAAGACTACCTGAAGCTTCA CAGAGTG ATTTATCAGCAAATTATCCAGACCTACCTG-3′, reverse primer: 5′-CAGGTAGGTCTGGATAATTTGCTGATAAAT CACTCTG TGAAGCTTCAGGTAGTCTTCTTC-3′) were generated using a QuikChange Site-Directed Mutagenesis Kit (Stratagene). Immunoprecipitation and immunoblotting For the immunoprecipitation experiment, cells were lysed with TAP buffer (25 mM Tris (pH 7.4), 140 mM NaCl, 0.5% NP-40, 10 mM NaF, 1 mM dithiothreitol (DTT), 1 mM phenylmethylsulphonyl fluoride , 1 mM EDTA, 1 mM Na 3 VO 4 , 1 mM β-glycerophosphate, 10% glycerol and 0.2% protease inhibitor cocktail) and incubated with rabbit-IgG (Jackson Laboratory) or anti-FLAG M2 affinity gel (Sigma-Aldrich) at 4 °C. The primary antibodies were purchased from commercial sources as follows: NCAPG2 (Novus Biological, 1/1,000), PLK1 (Novus Biological, 1/1,000), BubR1 (BD Biosciences, 1/1,000), β-actin (Sigma-Aldrich, 1/5,000) and CREST (ImmunoVision, 1/1,000). BubR1 676 antibodies(1/10,000) were prepared as previously reported [25] . Full blots are shown in Supplementary Fig. 6 . Expression and purification of PBD of PLK1 The human PLK1–PBD (371–594) was amplified using PCR and cloned into the pGEX6p-1 vector using the EcoRI and XhoI restriction enzyme sites. The protein was overexpressed in E. coli Rosetta2(DE3)pLysS cells (Novagen). The cells were grown at 37 °C in 3 l of Terrific Broth medium to an OD600 of 0.6, and recombinant protein expression was induced with 0.1 mM isopropyl β-D-thiogalactopyranoside (IPTG) at 20 °C. The cells were further grown at 20 °C for 20 h after IPTG induction. The purification methods were similar to methods that have been previously reported [36] . The purified protein was concentrated to 6 mg ml −1 and used for the fluorescence polarization binding assay or for crystal screening. Crystallization and structure determination The purified PBD and 5-mer 1010pT peptide (Ac-VLSpTL-NH 2 ; 5 mM final concentration) were mixed and stored on ice for an hour before the crystallization trial. The crystals of the PLK1–PBD in complex with the 1010pT peptide were obtained using the sitting drop vapour diffusion method. Crystals were grown in a reservoir solution of 200 mM potassium iodide, 100 mM MES (pH 6.5) and 25% (v/v) PEG 4000. X-ray diffraction data were collected using an ADSC Q315r CCD detector at Pohang Light Source, Korea. Intensity data were processed and scaled using the program HKL2000 (ref. 53 ). The structure was determined by molecular replacement using the programme Phaser [54] , and the model was refined using the programme Phenix [55] . Manual model building was performed using the programme Coot [56] . Fluorescence polarization binding assay for the PBD For the fluorescence polarization binding assay, fluorescein isothiocyanate-labelled 1010pT (GVLSpTLI) or 1010T (GVLSTLI) peptide was mixed with purified PBD and incubated in a buffer containing 10 mM HEPES (pH 7.5), 50 mM NaCl, 1 mM EDTA, 1 mM DTT and 0.0025% (v/v) Tween 20. The final protein concentrations ranged from 0 to 4 μM, and the final peptide concentration was 10 nM. Fluorescence polarization was analysed 30 min after mixing the peptide and proteins in a 96-well plate using a VERSAmax microplate reader (Molecular Devices). Binding curves were fitted using the GraphPad Prism software (GraphPad Software). Accession codes: The coordinates for the PBD of the PLK1-1010pT peptide complex have been deposited in the Protein Data Bank under accession code 4O9W . How to cite this article: Kim, J. H. et al. The condensin component NCAPG2 regulates microtubule–kinetochore attachment through recruitment of Polo-like kinase 1 to kinetochores. Nat. Commun. 5:4588 doi: 10.1038/ncomms5588 (2014).